Direct C–H difluoromethylation of heterocycles via organic photoredox catalysis The discovery of modern medicine relies on the sustainable development of synthetic methodologies to meet the needs associated with drug molecular design. Heterocycles containing difluoromethyl groups are an emerging but scarcely investigated class of organofluoro molecules with potential applications in pharmaceutical, agricultural and material science. Herein, we developed an organophotocatalytic direct difluoromethylation of heterocycles using O 2 as a green oxidant. The C–H oxidative difluoromethylation obviates the need for pre-functionalization of the substrates, metals and additives. The operationally straightforward method enriches the efficient synthesis of many difluoromethylated heterocycles in moderate to excellent yields. The direct difluoromethylation of pharmaceutical moleculars demonstrates the practicability of this methodology to late-stage drug development. Moreover, 2′-deoxy-5-difluoromethyluridine (F 2 TDR) exhibits promising activity against some cancer cell lines, indicating that the difluoromethylation methodology might provide assistance for drug discovery. Organofluoro compounds are widely used in the fields of pharmaceutical, agricultural, and material science [1] , [2] , [3] . The introduction of fluorine atoms or fluorine-containing groups into the framework of organic molecules often changes the physicochemical properties or biological activities of compounds [4] , [5] , [6] , [7] , [8] , and has become an essential topic for chemists. During the past few decades, much attention has been focused on the synthesis of fluorinated [9] , [10] , [11] , [12] and trifluoromethylated molecules [13] , [14] , [15] , [16] , [17] , [18] , [19] . On the other hand, the difluoromethyl is also a critical fluorinated functional group due to its use as a lipophilic hydrogen bond donor. In addition, CF 2 H group can be considered as the isostere of a thiol, a hydroxyl, and an amide, which brings out its potential value in drug development with novel scaffold [20] , [21] . However, unlike well-developed synthesis of fluorinated and trifluoromethylated compounds, the construction of difluoromethylated substances [22] , [23] , [24] , [25] , [26] , [27] , especially for difluoromethylated heterocycles, which widely exist in bioactive molecules (Fig. 1a ), has been less explored. The traditional strategies for the synthesis of difluoromethylated heterocycles include deoxyfluorination of aldehydes [28] , difluorination of benzylic C−H bonds [29] , [30] , decarbonylation/decarboxylation difluoromethylation [31] , [32] , cycloaddition reactions [24] , [33] , [34] , and conversion of CF 2 R containing heterocycles precursors [35] , [36] . However, these above-mentioned methods need expensive and toxic fluorinating agents, harsh reaction conditions, and are limited in functional group compatibility. Recently, difluoromethylation of heteroaromatic compounds catalyzed by transition metals [37] , such as copper, palladium, nickel, has been developed. However, most of these approaches depend on preactivation of substrates (i.e., aryl halides [38] , [39] , [40] , [41] , [42] , aryl boronic acids [43] , [44] , [45] , arylzincs [46] , arenediazonium salts [47] ). Fig. 1: Construction of CF 2 H-containing heterocycles. a Examples of CF 2 H- bioactive molecules. b TBHP promoted direct difluoromethylation of heterocycles. c High-energy light promoted direct difluoromethylation of heterocycles. d Ag and K 2 S 2 O 8 co-catalyzed direct difluoromethylation of heterocycles. e Cu and PQ co-catalyzed direct difluoromethylation of heterocycles. f Organic photoredox catalysis triggered direct difluoromethylation of heterocycles. Full size image The radical-based difluoromethylation method has been developed as an advantageous synthetic strategy for the construction of difluoromethylated heterocycles. The pioneering work was reported by Baran and co-workers (Fig. 1b ), in which they developed a new difluoromethylated reagent Zn(SO 2 CF 2 H) 2 (DFMS) that can effectively release CF 2 H radical in the presence of tert -butyl hydroperoxide (TBHP) as a stoichiometric oxidant [48] . Sakamoto et al. presented a photolytic direct C–H difluoromethylation of heterocycles using hypervalent iodine(III) reagents that contain difluoroacetoxy ligands (Fig. 1c ) [49] . Shortly afterward, Tung et al. developed direct difluoromethylation of heterocycles using difluoroacetic acid as CF 2 H radical precursors via transition metal catalysis (Fig. 1d ) [50] . In 2018, Zhu et al. reported a new strategy through the copper-mediated C−H oxidative difluoromethylation of heterocycles with TMSCF 2 H (Fig. 1e ) [51] . It should be noted that these protocols of direct difluoromethylation of heterocycles need either expensive/toxic metal catalysts or external oxidants and strictly inert conditions, which narrow the functional group tolerance and limit the substrate scope. During the submission of this manuscript, Duan and Xia reported an efficient photocatalytic strategy for C–H perfluoroalkylation of quinoxalinones under aerobic oxidation conditions, however, the corresponding difluoromethylation has not been reported [52] . Therefore, it is highly desirable to develop new approaches to achieve direct C–H difluoromethylation of heterocycles, which can overcome the above-mentioned defects and avoid the safety problems with stoichiometric oxidant at a larger scale. In the past decade, visible-light catalysis has attracted extensive attention, by which highly active radical species generated under mild conditions can be involved in various chemical bond formation [53] , [54] , [55] , [56] , [57] , [58] , [59] . Notably, organic dyes are cheaper and more reliable than expensive metal photoredox catalysts in many valuable reactions [55] , [56] , [59] . In this study, we focus our attention on developing an straightforward and practical method for difluoromethylation reactions using the inexpensive, commercially available, and user friendly Hu’s reagent sodium difluoromethane sulfonate (CF 2 HSO 2 Na) as the difluoromethyl radical precursor [60] under mild conditions. This protocol combines organic photocatalysis with green air oxidant for the difluoromethylation of many categories of heterocycles. Notably, the difluoromethylation product 2′-deoxy-5-difluoromethyluridine (F 2 TDR) commendably inhibits the proliferation of cancer cells, such as HCT116, HepG-2, and MCF-7 (Fig. 1f ). Investigation of the reaction conditions We started our investigation by the model reaction of 1-methyl quinoxolin-2-one 1a with CF 2 HSO 2 Na 2 as a fluorine source and eosin Y as a photocatalyst in DMSO at room temperature under green LEDs irradiation. 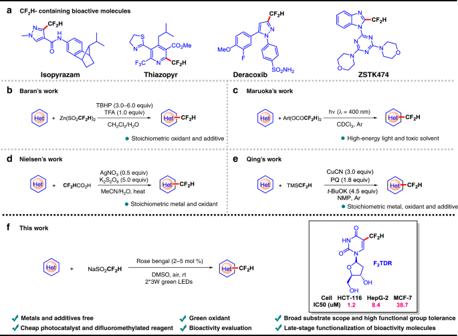Fig. 1: Construction of CF2H-containing heterocycles. aExamples of CF2H- bioactive molecules.bTBHP promoted direct difluoromethylation of heterocycles.cHigh-energy light promoted direct difluoromethylation of heterocycles.dAg and K2S2O8co-catalyzed direct difluoromethylation of heterocycles.eCu and PQ co-catalyzed direct difluoromethylation of heterocycles.fOrganic photoredox catalysis triggered direct difluoromethylation of heterocycles. To our delight, the difluoromethylation product 3a was obtained in 64% yield (Table 1 , entry 1). Then, different photocatalysts were examined (Table 1 , entries 2–8), in which rose bengal (RB) was the best one, providing 3a in 72% yield in 12 h. After identifying the optimal photocatalyst, we found that DMSO was the best reaction media through solvent screening (Table 1 , entries 2 and 9–16). The yield of product reduced obviously when the loading of the photocatalyst was further decreased to 1 mol% (Table 1 , entry 17). Control experiments indicated that photocatalyst and green light source were both essential for the reaction efficiency (Table 1 , entries 18 and 19). Table 1 Reaction optimization a,b . Full size table Scope of quinoxalin-2( 1H )-ones on the phenyl ring With the optimal reaction conditions in hand, the substrate scope of various quinoxalin-2(1 H )-ones was then investigated. As exhibited in Fig. 2 , the reactions worked well with a range of substituted quinoxalin-2(1 H )-ones bearing either electron-donating or -withdrawing substituents (methyl, fluoro, chloro, bromo, methoxy, nitro, and naphthyl), giving the desired difluoromethylation products 3a – 3j in moderate to good yields. To highlight the utility of this transformation, a variety of N -substituted quinoxalin-2(1 H )-ones ( 1k−1n ) were also tested. As a result, all the N -substituted quinoxalin-2(1 H )-ones are compatible with the reaction, furnishing the expected products 3k–3n in 34–73% yields. Notably, N -unsubstituted quinoxalin-2(1 H )-one also proceeded smoothly, delivering the desired product 3o in 87% yield. Fig. 2: Substrate scope of quinoxalin-2(1 H )-ones. Reaction conditions: 1 (0.2 mmol), CF 2 HSO 2 Na 2 (0.4 mmol), rose bengal (2 mol%) in 1 mL DMSO under two 3 W green LEDs irradiation at room temperature. Isolated yields based on 1 . Full size image Scope of heteroaromatics To further extend the scope of this methodology, some other heteroaromatic substrates were investigated (Fig. 3 ). A wide range of five- and six-membered difluoromethylated heteroarenes, such as pyrazines ( 5a and 5b ), quinoxalines ( 5c and 5d) , pyrrole ( 5e ), imidazoles ( 5f and 5g ), thiophene ( 5i ), pyridines ( 5j ), thiadiazole ( 5k ), indoles ( 5l and 5m ), RNA-based dimethyluracils ( 5n and 5o ), quinoline ( 5p ), purine derivatives ( 5q and 5r ), and pyrimidine ( 5 s ), provided final products with good yields. Several heteroarenes with potentially sensitive functional groups (OH, NH 2 , or CHO) ( 5a , 5k , and 6j ) that are barely reported in the previous study [48] , [49] , [50] , [51] are also compatible with this difluoromethylation strategy. Moreover, this direct C–H difluoromethylation method also suitable for some arenes ( 5t and 6j ). Fig. 3: Substrate scope of heteroaromatics. Reaction conditions: 4 (0.1 mmol), CF 2 HSO 2 Na 2 (0.4 mmol), rose bengal (5 mol.%) in 1 mL DMSO under two 3 W green LEDs irradiation at room temperature. Isolated yields based on 4 . b With CF 2 HSO 2 Na 2 (0.4 mmol), rose bengal (2 mol%) in 1 mL DMSO. Full size image Scope of bioactive molecules The methodology can also be applied to late-stage functionalization of complex nitrogen-containing bioactive molecules (Fig. 4 ). For example, the modification of caffeine and its derivatives delivers the desired difluoromethylated products 6a – 6c in 38–74% yields. In addition, deoxyuridine, uridine, and 2′-fluoro-2′-deoxyuridine, which have free OH group as well as amide group, could tolerate this difluoromethylation reaction, leading to 6d – 6f in 57–81% yields. Furthermore, melatonin, allopurinol, and uracil, which bear free secondary N–H groups, furnished the difluoromethylation reaction with moderate to good yields ( 6g , 6h , and 6l ). Moreover, some other bioactive heteroarene substrates, such as voriconazole, flavorant, metyrapone, and sulfonylureas, can also proceed well with the reaction, giving the difluoromethylated products 6i , 6j , 6k , and 6m in acceptable yields. Fig. 4: Substrate scope of bioactive molecules. Reaction conditions: 4 (0.1 mmol), CF 2 HSO 2 Na 2 (0.4 mmol), rose bengal (5 mol%) in 1 mL DMSO under two 3 W green LEDs irradiation at room temperature. Isolated yields based on 4 . b With CF 2 HSO 2 Na 2 (0.4 mmol), rose bengal (2 mol%) in 1 mL DMSO. c Large scale with 2 mmol heteroarenes. d The minor regioisomeric position is labeled with the respective carbon atom number. Full size image Site-selectivity study The substrate scope results of Figs. 2 – 4 show that most of the difluoromethylation occurs on the C2–H bond adjacent to the heteroatom. Some heterocycle substrates bearing more than one radical attacked carbon center were also examined (Fig. 5 ). As a result, the unsubstituted indole substrate 7 gave the major product at the C2 position in 54% yield with 10:1 regioselectivity. The 5-nitro-substituted indole substrate 9 can obtain a single regioselective difluoromethylation product 10 with 71% yield. When 4-chloro-7H-pyrrolo[2,3-d] pyrimidine was used as substrate, the reaction furnish the mixture of product 12 (C2/C6 = 5:1) in 46% yield. Notably, other electron-rich heteroarenes (benzofuran 13 and thianaphthene 15 ), which have not been investigated as substrates in previous reported radical difluoromethylation reactions [48] , [49] , [50] , also exhibited good reaction efficiency, producing the difluoromethylation products 14 and 16 in 92% and 65% yield, respectively. Unfortunately, other types of heteroarenes, including phenanthroline, 1,3,5-triazine, and thiazone, are not ideal substrates in this difluoromethylation reaction (Supplementary Fig. 2 ). Fig. 5: Site-selectivity study. a Regioselectivity for indoles. b Regioselectivity for 4-chloro-7H-pyrrolo[2,3-d] pyrimidine. c Regioselectivity for benzofuran. d Regioselectivity for thianaphthene. 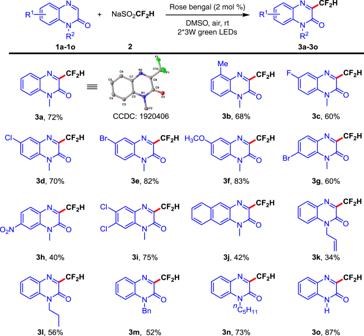Fig. 2: Substrate scope of quinoxalin-2(1H)-ones. Reaction conditions:1(0.2 mmol), CF2HSO2Na2(0.4 mmol), rose bengal (2 mol%) in 1 mL DMSO under two 3 W green LEDs irradiation at room temperature. Isolated yields based on1. Reaction conditions: heterocycles (0.1 mmol), CF 2 HSO 2 Na 2 (0.4 mmol), rose bengal (5 mol%) in 1 mL DMSO under two 3 W green LEDs irradiation at room temperature. Isolated yields based on heterocycles. b The minor regioisomeric position is labeled with the respective carbon atom number. Full size image Synthetic applications To evaluate the synthetic potential of this methodology, sunlight-driven experiment was performed. When the reaction was conducted under sunlight irradiation, the desired product 3a was obtained in 68% yield (Fig. 6a ). Furthermore, a slight reduction of yields with large scale preparation of 6d and 6g also prove the practicability of this difluoromethylation strategy (Fig. 4 , yields in parentheses for 6d and 6g ). We further explored the potential application of the synthesized difluoromethylated product in medicinal chemistry. The F 2 TDR 6d has a similar structure to the trifluridine, which has been approved by FDA for the treatment of adult patients with metastatic colorectal cancer (for details, see https://www.drugbank.ca/drugs/DB00432 ). Therefore, we selected four tumor cell lines to evaluate the inhibitory activities of 6d , and made the comparison of the result with trifluridine. As shown in Fig. 6b , 6d higher tumor cell inhibitory capability than the trifluridine with relatively low IC 50 values. Notably, the IC 50 values of 6d against HCT116 and HepG-2 cells reach low micromolar level, which are about 57- and 6-fold lower than that of trifluridine, respectively. The improvement of antitumor activity indicates the practicality of this difluoromethylation methodology and the potential in the field of discovery of active drug molecules. Fig. 6: Synthetic applications. a The reactions were carried out with 4 (0.1 mmol), CF 2 HSO 2 Na 2 (0.2 mmol), rose bengal (2 mol%) in 1 mL DMSO under sunlight irradiation at room temperature. b Cytotoxicity of compounds. i MCF-7 (human breast adenocarcinoma cells), ii HepG-2 (human liver hepatocellular carcinoma cells), iii HCT116 (human colorectal cancer cells), and iv Hela (human cervical carcinoma cells) were treated with various concentrations of each compound for 72 h. Cell death was then measured by using a CCK-8 assays ( n = 5, mean ± SD). Full size image Mechanistic investigations To gain insights into the current studied reaction, control experiments were conducted. When a radical scavenger, 2,2,6,6-tetramethyl-1-piperidinyloxy (TEMPO) or 1,1-diphenylethylene (Fig. 7a, b ) was existing in the mixture containing 1a and CF 2 HSO 2 Na, the reaction was completely suppressed, while the radical intermediate was detected by ESI-HRMS (Supplementary Fig. 5 ), indicating the existence of CF 2 H radical. When the reaction was carried out under inert atmosphere (Fig. 7c ), the formation of 3a was completely inhibited, revealing that oxygen is crucial for the reaction. In situ 1 H NMR experiment demonstrated that hydrogen peroxide (H 2 O 2 ) does not form after irradiation of the reaction mixture in DMSO- d 6 for 12 h under the optimized reaction condition. In addition, the observed water peak (H 2 O) growth indicating that the oxygen was eventually converted to H 2 O rather than H 2 O 2 (Supplementary Figs. 6 and 7 ). The generated H 2 O 2 could participate in the catalytic cycle and ultimately converted to H 2 O as the byproduct [61] . These experimental results illustrated an available radical pathway. Moreover, we also conducted the light/dark experiment. As shown in Fig. 7 , the desired product 3a formed only under continuous irradiation, which ruled out the possibility of a radical chain propagation. On the basis of our experimental observations and previous studies [59] , a possible mechanism was proposed (Fig. 7e ). 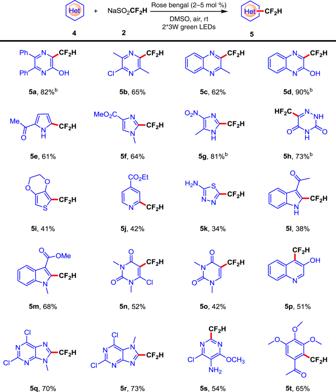Fig. 3: Substrate scope of heteroaromatics. Reaction conditions:4(0.1 mmol), CF2HSO2Na2(0.4 mmol), rose bengal (5 mol.%) in 1 mL DMSO under two 3 W green LEDs irradiation at room temperature. Isolated yields based on4.bWith CF2HSO2Na2(0.4 mmol), rose bengal (2 mol%) in 1 mL DMSO. Upon absorption of visible light, the photocatalyst RB is excited into RB* ( E red = 0.99 V vs SCE) and a single electron is transferred from CF 2 HSO 2 Na [62] ( E = 0.59 V vs SCE) to RB*, which affords CF 2 H radical and generates an RB •− radical anion. The photoredox cycle is completed by the molecular oxygen oxidation of RB •− , giving RB and O 2 •− . After that, addition of CF 2 H radical to 1a occurs, leading to intermediate A , which undergoes a 1,2-H shift to generate carbon radical intermediate B . The intermediate B loses a hydrogen atom to O 2 •− to furnish the desired product 3a . Fig. 7: Mechanistic investigations. 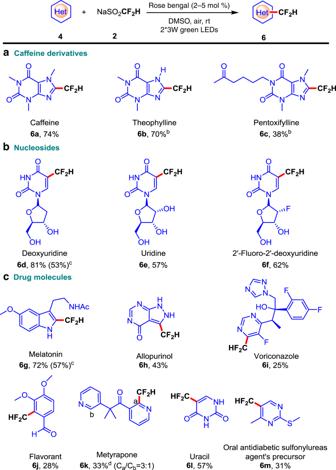Fig. 4: Substrate scope of bioactive molecules. Reaction conditions:4(0.1 mmol), CF2HSO2Na2(0.4 mmol), rose bengal (5 mol%) in 1 mL DMSO under two 3 W green LEDs irradiation at room temperature. Isolated yields based on4.bWith CF2HSO2Na2(0.4 mmol), rose bengal (2 mol%) in 1 mL DMSO.cLarge scale with 2 mmol heteroarenes.dThe minor regioisomeric position is labeled with the respective carbon atom number. a Investigation on the effect of TEMPO. b Radical trapping with 1,1-diphenylethylene. c Investigation on the effect of oxygen. d Light/dark experiment. e Proposed reaction mechanism. Full size image In summary, we have achieved a visible-light triggered direct C–H difluoromethylation of heterocycles by using commercially available and inexpensive sodium difluoromethane sulfonate as CF 2 H radical source. The process is  under mild conditions using O 2 as a green oxidant and without using  metal additive. Furthermore, we also use this highly efficient methodology for direct difluoromethylation of some nitrogen-containing biological and pharmaceutical active molecules. In addition, the bioactivity evaluation of a representative difluoromethylation product 2′-deoxy-5-difluoromethyluridine ( 6d ) exhibited promising activity against cancer cell lines. We expect this simple protocol to be of broad utility for the development of new drugs. 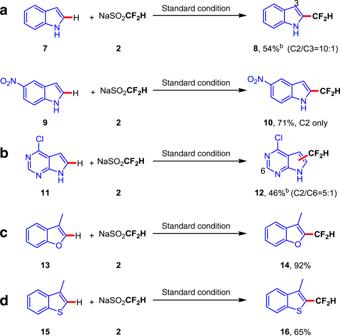Fig. 5: Site-selectivity study. aRegioselectivity for indoles.bRegioselectivity for 4-chloro-7H-pyrrolo[2,3-d] pyrimidine.cRegioselectivity for benzofuran.dRegioselectivity for thianaphthene. Reaction conditions: heterocycles (0.1 mmol), CF2HSO2Na2(0.4 mmol), rose bengal (5 mol%) in 1 mL DMSO under two 3 W green LEDs irradiation at room temperature. Isolated yields based on heterocycles.bThe minor regioisomeric position is labeled with the respective carbon atom number. Further synthetic applications and bioactivity tests are ongoing. Procedure for difluoromethylation of quinoxalin-2(1 H )-ones To a 10 mL Schlenk tube equipped with a magnetic stir bar added quinoxalin-2(1 H )-ones 1 (0.2 mmol), CF 2 HSO 2 Na 2 (0.4 mmol), and RB (0.004 mmol, 2 mol.%) in DMSO (1.0 mL). Then the mixture was stirred and irradiated by two 3 W green LEDs at room temperature for 12 h. The residue was added water (10 mL) and extracted with ethyl acetate (5 mL × 3). The combined organic phase was dried over Na 2 SO 4 . The resulting crude residue was purified via column chromatography on silica gel to afford desired products. Procedure for difluoromethylation of other heterocycles To a 10 mL Schlenk tube equipped with a magnetic stir bar added heteroarenes 4 (0.1 mmol), CF 2 HSO 2 Na 2 (0.4 mmol), and RB (0.002–0.005 mmol, 2–5 mol.%) in DMSO (1.0 mL). 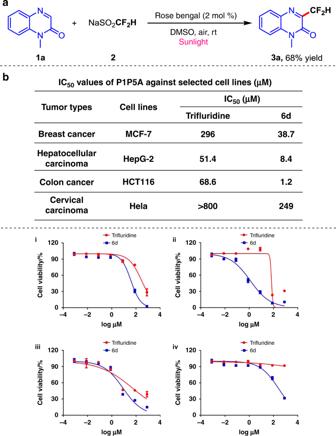Fig. 6: Synthetic applications. aThe reactions were carried out with4(0.1 mmol), CF2HSO2Na2(0.2 mmol), rose bengal (2 mol%) in 1 mL DMSO under sunlight irradiation at room temperature.bCytotoxicity of compounds. i MCF-7 (human breast adenocarcinoma cells), ii HepG-2 (human liver hepatocellular carcinoma cells), iii HCT116 (human colorectal cancer cells), and iv Hela (human cervical carcinoma cells) were treated with various concentrations of each compound for 72 h. Cell death was then measured by using a CCK-8 assays (n= 5, mean ± SD). 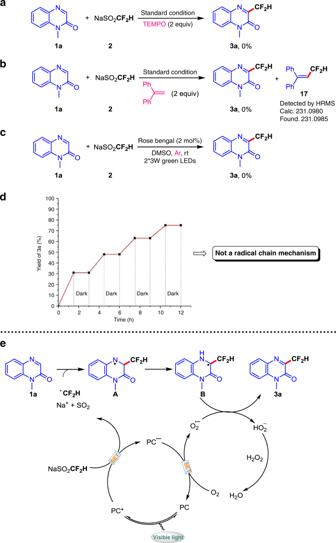Fig. 7: Mechanistic investigations. aInvestigation on the effect of TEMPO.bRadical trapping with 1,1-diphenylethylene.cInvestigation on the effect of oxygen.dLight/dark experiment.eProposed reaction mechanism. Then the mixture was stirred and irradiated by two 3 W green LEDs at room temperature for 24 h. The residue was added water (10 mL) and extracted with ethyl acetate (5 mL × 3). The combined organic phase was dried over Na 2 SO 4 . The resulting crude residue was purified via column chromatography on silica gel to afford desired products.